Treatment of acute lung injury by targeting MG53-mediated cell membrane repair Injury to lung epithelial cells has a role in multiple lung diseases. We previously identified mitsugumin 53 (MG53) as a component of the cell membrane repair machinery in striated muscle cells. Here we show that MG53 also has a physiological role in the lung and may be used as a treatment in animal models of acute lung injury. Mice lacking MG53 show increased susceptibility to ischaemia–reperfusion and overventilation-induced injury to the lung when compared with wild-type mice. Extracellular application of recombinant human MG53 (rhMG53) protein protects cultured lung epithelial cells against anoxia/reoxygenation-induced injuries. Intravenous delivery or inhalation of rhMG53 reduces symptoms in rodent models of acute lung injury and emphysema. Repetitive administration of rhMG53 improves pulmonary structure associated with chronic lung injury in mice. Our data indicate a physiological function for MG53 in the lung and suggest that targeting membrane repair may be an effective means for treatment or prevention of lung diseases. Living cells in most organs in the human body, including the skin, gastrointestinal tract, striated muscles and lungs are subjected to constant mechanical stress. Plasma membrane disruptions often occur as a result, causing release of intracellular contents and inflammatory mediators, and leading to disruption of cellular function and even cell death. In response to loss of cells by these insults, tissues can compensate either by proliferation to replace injured cells or minimize the death of individual cells through repair mechanisms to restore the integrity of cell membrane [1] , [2] , [3] , [4] . Such repair mechanisms are of particular importance to cells with low proliferative capacity. Our previous studies identified mitsugumin 53 (MG53), a member of the tripartite motif (TRIM) family protein, as an essential component of the cell membrane repair machinery in striated muscles [5] , [6] , [7] , [8] , [9] , [10] , [11] . Native MG53 functions in vesicle trafficking and allows for nucleation of intracellular vesicles at sites of membrane disruption [5] . Knockout mice for mg53 ( mg53−/− ) display defective membrane repair in striated muscles that leads to progressive skeletal myopathy and increased vulnerability of cardiomyocytes to membrane injury following ischaemia–reperfusion (I/R) injury [5] , [7] , [9] , [10] . Injury to lung epithelial cells has been implicated in the pathogenesis and progression of multiple lung diseases [12] , [13] . I/R-induced lung injury is a common cause of morbidity and mortality under a wide range of medical conditions, such as lung and/or heart organ transplantation, acute pulmonary embolism, pulmonary thrombosis and cardiopulmonary bypass surgery [14] , [15] , [16] , [17] . Various pathological stresses such as pneumonia, sepsis, trauma and blood transfusion can also result in acute lung injury (ALI) and acute respiratory distress syndrome [12] , [18] . The major clinical manifestations of ALI, including inflammatory cell infiltration, arterial hypoxaemia and pulmonary oedema, are direct consequences of the disrupted airway and alveolar barrier function. Thus, effective ALI treatment requires resolution of alveolar oedema and restoration of epithelial and endothelial barrier integrity. A few approaches for ALI have been developed to address these aspects, including low tidal volume ventilation and fluid-conservative therapy and anti-inflammation [13] . However, because of the limited knowledge of the cell biology for membrane repair in lung physiology, direct therapeutic approaches for ALI that target membrane repair in airway and alveolar epithelial cells has not been well developed. Although our previously published studies have focused on the cell membrane repair function for MG53 in skeletal and cardiac muscles, here we present evidence that MG53 is also expressed in alveolar cells of the lung tissue. Compared with wild-type mice, mg53−/− mice show increased susceptibility to damage following I/R injury and overventilation of the lung. We also tested the therapeutic effect of the recombinant human MG53 (rhMG53) protein [19] in treating damage to the lung, using in vitro and in vivo models of acute and chronic lung injury. Our data suggest that targeting MG53 function could represent an effective means for restoration of barrier function and integrity of the airway and alveolar epithelial cells during ALI. MG53 protein is expressed in lung tissue The mg53 gene was originally cloned from skeletal muscle using an immuno-proteomics approach [20] . Biochemical studies showed that MG53 protein is enriched in striated muscles [5] , [7] , [21] . Here we tested whether MG53 protein is also expressed in the lung. Western blotting showed that MG53 could only be detected in lysates of lung tissue derived from the wild-type mice, but not in the mg53−/− lung homogenate ( Fig. 1a and Supplementary Fig. 1 ). Quantitative assessment revealed that the level of MG53 protein in the lung tissue is ~5% of that in skeletal muscle. 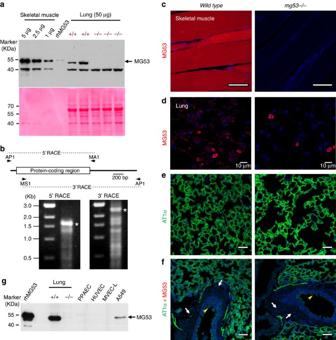Figure 1: Expression of MG53 in lung tissue. (a) Homogenates of lung tissue derived from the wild-type andmg53−/−mice were used for western blotting for the detection of MG53. rhMG53 (0.1 ng) was used as positive control. For comparative purpose, the content of MG53 in skeletal muscle was assayed at different concentrations of muscle tissues. Ponceau S staining reveals differential loading of the skeletal muscle and lung tissues. A nonspecific 40-kDa protein was also recognized by our custom-made anti-MG53 antibody. The uncropped western blotting images are shown inSupplementary Fig 1. (b) Characterization of lungmg53transcripts by RACE cDNA amplification. The cDNA amplification strategy is illustrated in the upper panel. A mouse lung cDNA preparation was amplified using AP1 and MA1 primers in the 5′-RACE reaction or using MS1 and AP1 primers in the 3′-RACE reaction. Amplified cDNA products in each RACE reaction were analysed in agarose electrophoresis as shown in the lower panel. Putative full-length cDNAs marked with asterisks were extracted from agarose gels and subcloned into a plasmid vector for sequencing. The protein-coding sequence of the amplified lungmg53cDNAs was identical to that of musclemg53cDNAs determined in our previous study. (c) Immunohistochemical (IHC) staining with an anti-MG53 antibody revealed high level of MG53 in wild-type skeletal muscle, which is absent in themg53−/−muscle. (d–f) IHC staining of lung tissues derived from wild-type (left panels) ormg53−/−mice (right panels). Compared with skeletal muscle, low level of MG53 could be detected in the lung (d). Background staining in themg53−/−lung probably reflects autofluorescence of capillary cells or nonspecific activity of the anti-MG53 antibody (see the 40-kDa band ina). The MG53 expression pattern in wild-type lung matches to that of AT1α, a type I alveolar cell marker (e). The MG53 and AT1α (type 1a angiotensin II receptor) (anti-AT1α, Novus Biologicals NB600-1015) stainings (d,e) were shown separately to better indicate the localization of MG53 due to its low expression in alveolar cells. The cross-section of bronchioles revealed negative staining for MG53 in both airway smooth muscle layer (arrow) and the neighbouring ciliated endothelial lining of the airway lumen (arrow head) (f). Scale bars, 50 μm. (g) Immunoblotting of MG53 with lysates from mouse lung tissues, and cells derived from A549, human pulmonary artery endothelial cell (PPAEC), human lung microvascular endothelial cell (MVEC-L) and human umbilical vein endothelial cell (HUVEC; 50 μg per lane). rhMG5 (1 ng) served as a positive control for the immunoblotting. Figure 1: Expression of MG53 in lung tissue. ( a ) Homogenates of lung tissue derived from the wild-type and mg53−/− mice were used for western blotting for the detection of MG53. rhMG53 (0.1 ng) was used as positive control. For comparative purpose, the content of MG53 in skeletal muscle was assayed at different concentrations of muscle tissues. Ponceau S staining reveals differential loading of the skeletal muscle and lung tissues. A nonspecific 40-kDa protein was also recognized by our custom-made anti-MG53 antibody. The uncropped western blotting images are shown in Supplementary Fig 1 . ( b ) Characterization of lung mg53 transcripts by RACE cDNA amplification. The cDNA amplification strategy is illustrated in the upper panel. A mouse lung cDNA preparation was amplified using AP1 and MA1 primers in the 5′-RACE reaction or using MS1 and AP1 primers in the 3′-RACE reaction. Amplified cDNA products in each RACE reaction were analysed in agarose electrophoresis as shown in the lower panel. Putative full-length cDNAs marked with asterisks were extracted from agarose gels and subcloned into a plasmid vector for sequencing. The protein-coding sequence of the amplified lung mg53 cDNAs was identical to that of muscle mg53 cDNAs determined in our previous study. ( c ) Immunohistochemical (IHC) staining with an anti-MG53 antibody revealed high level of MG53 in wild-type skeletal muscle, which is absent in the mg53−/− muscle. ( d – f ) IHC staining of lung tissues derived from wild-type (left panels) or mg53−/− mice (right panels). Compared with skeletal muscle, low level of MG53 could be detected in the lung ( d ). Background staining in the mg53−/− lung probably reflects autofluorescence of capillary cells or nonspecific activity of the anti-MG53 antibody (see the 40-kDa band in a ). The MG53 expression pattern in wild-type lung matches to that of AT1α, a type I alveolar cell marker ( e ). The MG53 and AT1α (type 1a angiotensin II receptor) (anti-AT1α, Novus Biologicals NB600-1015) stainings ( d , e ) were shown separately to better indicate the localization of MG53 due to its low expression in alveolar cells. The cross-section of bronchioles revealed negative staining for MG53 in both airway smooth muscle layer (arrow) and the neighbouring ciliated endothelial lining of the airway lumen (arrow head) ( f ). Scale bars, 50 μm. ( g ) Immunoblotting of MG53 with lysates from mouse lung tissues, and cells derived from A549, human pulmonary artery endothelial cell (PPAEC), human lung microvascular endothelial cell (MVEC-L) and human umbilical vein endothelial cell (HUVEC; 50 μg per lane). rhMG5 (1 ng) served as a positive control for the immunoblotting. Full size image We consistently observed a slight mobility shift of MG53 from the lung tissue compared with that in the muscle tissue and the rhMG53 protein obtained from Escherichia coli fermentation [19] ( Fig. 1a ). To investigate whether this is due to splice variation among different tissues, rapid amplification of complementary DNA end (RACE) analysis was performed with a mouse lung cDNA library. Both 5′-RACE and 3′-RACE produced cDNA coding sequences for MG53 ( Fig. 1b ). Sequencing of multiple clones from the 5′-RACE and 3′-RACE reactions revealed identical mg53 sequences in lung and muscle tissue ( Supplementary Table 1 ). These studies indicate that the full-length mRNA for MG53 is expressed in the lung, thus potential post-translational modification/processing mechanisms may be responsible for the mobility shift for MG53 observed in the lung tissue. Further studies will be required to understand this mechanism. Immunohistochemical staining with lung tissues derived from wild-type and mg53−/− mice was used to probe the cell-type-specific expression for MG53 in the lung. As shown in Fig. 1c , high level expression of MG53 was detected from the wild-type skeletal muscle but not from the mg53−/− skeletal muscle. Compared with skeletal muscle, lower level expression of MG53 was present in the alveolar epithelial cells ( Fig. 1d ). The distribution of MG53 was similar to that of AT1α, a specific cell marker for type I alveolar epithelial cells ( Fig. 1e ). These histological studies also indicated that MG53 is absent from smooth muscle and vascular endothelial cells ( Fig. 1f ). Because of the difficulty of isolating primary cultured type I and type II alveolar epithelial cells from mice, we performed immunoblotting with cultured adenocarcinoma human type II alveolar epithelial cells (A549), human lung microvascular endothelial cells, human pulmonary artery endothelial cells and human umbilical vein endothelial cells. As shown in Fig. 1g , endogenous MG53 could be detected in A549 cells, but not in endothelial cells. In a small portion of immunohistochemical staining with the pulmonary vessel wall, we observed a strong striation pattern of MG53 signal, which is present in the wild-type lung and absent from the mg53−/− lung (see Supplementary Fig. 2 ). Such MG53 signal probably originated from potential lung-resident cardiomyocytes, as a recent report by Krachlauer et al. [22] showed that the mouse and rat lung tissues contain unique patterns of venous cardiomyocytes. Taken together, our data suggest that MG53 is present in both type I and type II alveolar epithelial cells, but absent from endothelial cells. Knockout of MG53 exacerbates stress-induced lung injury The presence of MG53 in the lung tissue suggests the possibility of a lung phenotype in the mg53−/− mice. Histological analysis revealed pathological changes with lung derived from the mg53−/− mice under normal conditions. Haematoxylin–eosin staining showed enlarged alveolar space with the mg53−/− lung when compared with the wild-type littermates ( Fig. 2a ). This finding is consistent with the expression of MG53 in the alveolar epithelial cells, as the absence of MG53 may lead to defective alveolar structure in the mutant mice. 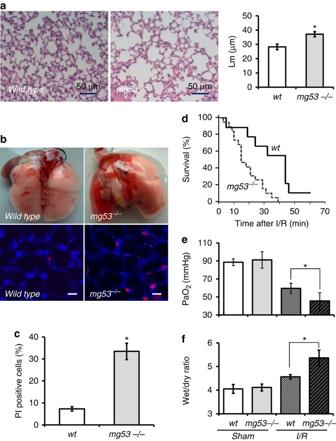Figure 2: Increased susceptibility of themg53−/−mice to overventilation and I/R-induced lung injury. (a) Haematoxylin and eosin staining of lung section derived from wild-type andmg53−/−mice under basal conditions. Mean linear intercept measurements (Lm) of alveolar spaces reveal significant difference between the wild-type andmg53−/−lung. (b) Representative images of wild-type andmg53−/−lung subjected to overventilation (upper panels). The subpleural lung images of wild-type andmg53−/−mice show PI+alveolus cells after overventilation (lower panels). Scale bar, 10 μm. (c) Quantification of PI+cells in the subplueral lung area after overventilation (n=4 for wild type;n=5 formg53−/−, *P<0.05, Student’st-test). (d). Survival rate ofmg53−/−and wild-type mice was recorded after I/R. The product limit (Kaplan–Meier) estimate of the cumulative survival was assessed with the log-rank test to evaluate for significant differences in survival (*P<0.05,n=19 formg53−/−mice andn=9 for wild type mice, Kaplan–Meier survival analysis (mean±s.e.m.). (e) Arterial blood samples were drawn from individual mice, the plasma PaO2concentrations were measured (*P<0.05 versus wild type,n=6 in each group, analysis of variance (ANOVA), mean±s.e.m.). (f) Lung oedema was measured as the wet/dry weight ratio of the excised lung from mice (*P<0.05 versus wild type,n=5, ANOVA). Animals receiving normal low-tidal ventilation without I/R were used as sham controls. Figure 2: Increased susceptibility of the mg53−/− mice to overventilation and I/R-induced lung injury. ( a ) Haematoxylin and eosin staining of lung section derived from wild-type and mg53−/− mice under basal conditions. Mean linear intercept measurements (Lm) of alveolar spaces reveal significant difference between the wild-type and mg53−/− lung. ( b ) Representative images of wild-type and mg53−/− lung subjected to overventilation (upper panels). The subpleural lung images of wild-type and mg53−/− mice show PI + alveolus cells after overventilation (lower panels). Scale bar, 10 μm. ( c ) Quantification of PI + cells in the subplueral lung area after overventilation ( n =4 for wild type; n =5 for mg53−/− , * P <0.05, Student’s t -test). ( d ). Survival rate of mg53−/− and wild-type mice was recorded after I/R. The product limit (Kaplan–Meier) estimate of the cumulative survival was assessed with the log-rank test to evaluate for significant differences in survival (* P <0.05, n =19 for mg53−/− mice and n =9 for wild type mice, Kaplan–Meier survival analysis (mean±s.e.m.). ( e ) Arterial blood samples were drawn from individual mice, the plasma PaO 2 concentrations were measured (* P <0.05 versus wild type, n =6 in each group, analysis of variance (ANOVA), mean±s.e.m.). ( f ) Lung oedema was measured as the wet/dry weight ratio of the excised lung from mice (* P <0.05 versus wild type, n =5, ANOVA). Animals receiving normal low-tidal ventilation without I/R were used as sham controls. Full size image We evaluated the susceptibility of these animals to overventilation-induced lung injury. For this purpose, wild-type and mg53−/− mice were ventilated at 30 ml kg −1 (tidal volume/body weight) to introduce acute stress to lung resident cells. Propidium iodide (PI) was injected into the right ventricle immediately after removal of injurious stress for labelling of necrotic cells. Wounded subpleural alveolus resident cells were then visualized by confocal microscopy [23] , [24] . As shown in Fig. 2b , 30-min overventilation did not produce measurable injury or changes in gross morphology to the wild-type lungs. In contrast, the same conditions in mg53−/− lungs resulted in large areas of haemorrhage and atelectasis, indicating increased susceptibility to injury of the lung tissue in the absence of MG53. Confocal imaging showed that a small percentage of alveolus resident cells were labelled by PI in the wild-type lung following overventilation ( Fig. 2b , lower left), which was consistent with previous studies by Gajic et al. [23] In the mg53−/− mice, the subpleural area of the lung displayed more PI-positive cells ( Fig. 2b , lower right), indicating the possibility of defective repair in these cells. Statistical analysis showed that following overventilation significantly more PI-positive cells appear in the mg53−/− lung compared with the wild-type lung ( Fig. 2c ). We also tested whether the absence of MG53 could alter the response of the lung following I/R-induced injury. For this purpose, littermates of wild-type and mg53−/− mice were subjected to 1 h ischaemia/1 h reperfusion by clamping of the left pulmonary artery and hilum to induce complete ischaemia and anoxia of the left lung. Compared with the wild-type controls, the mg53−/− mice had lower survival rate following I/R injury ( Fig. 2d ). Pulmonary function assessed by measurement of arterial blood gas showed that the PaO 2 in wild-type mice measured at 59.5±5.8 mm Hg, while it dropped to 45.5±9.2 mm Hg in mg53−/− mice ( n =6 in each, P -value<0.05, analysis of variance (ANOVA)) after I/R-induced lung injury ( Fig. 2e ). The wet/dry ratio of lungs harvested from wild-type mice was 4.56±0.09, whereas that in the mg53−/− mice was 5.37±0.33 ( n =6 in each, P <0.05, ANOVA) ( Fig. 2f ). These data suggest that systemic ablation of MG53 leads to increased susceptibility of the mice to I/R-induced injury to the lung. MG53 protects against injury in cultured lung epithelial cells We used cultured rat lung epithelial (RLE) cells to investigate the extent that MG53 participates in membrane repair of lung resident cells. The RLE cells were transfected with a fusion protein containing the green fluorescent protein (GFP) linked to the amino-terminal end of the mouse MG53 (GFP-MG53). GFP-MG53 in RLE cells localized primarily to the cytosol and plasma membrane ( Fig. 3a , left), a subcellular distribution similar to that observed in striated muscle [5] and other non-muscle cell types [19] . In response to injury caused by penetration of a micro-electrode into the plasma membrane, rapid translocation of GFP-MG53-labelled intracellular vesicles towards the acute injury site was observed ( Fig. 3a , right). This GFP-MG53 translocation to membrane injury sites in RLE cells is similar to those observed in C2C12, HEK293 and other cell types [5] , [19] . 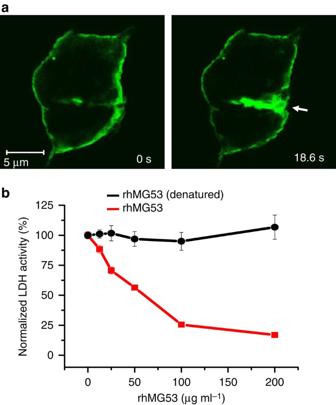Figure 3:In vitroassay with MG53 protection against injury to cultured RLE cells. (a) RLE cell transfected with GFP-MG53 show rapid translocation of GFP-MG53-containing intracellular vesicles towards the acute plasma membrane injury site following penetration of a microelectrode. Left panel—cell image taken immediately after injury; right panel—image taken 18.6 s after injury. Arrow shows the microelectrode injury site. Visualization of live cell imaging of the GFP-MG53 movement process can be found inSupplementary Movie 1. (b) RLE cells were treated with external rhMG53 or boiled rhMG53 (denatured control protein) in the cell culture medium and then exposed to mechanical membrane damage by glass beads. Membrane damage is measured by LDH release from cells. rhMG53 reduced LDH release due to mechanical damage and this protective effect is dose dependent,n=9–12 for each data point (mean±s.e.m.). Figure 3: In vitro assay with MG53 protection against injury to cultured RLE cells. ( a ) RLE cell transfected with GFP-MG53 show rapid translocation of GFP-MG53-containing intracellular vesicles towards the acute plasma membrane injury site following penetration of a microelectrode. Left panel—cell image taken immediately after injury; right panel—image taken 18.6 s after injury. Arrow shows the microelectrode injury site. Visualization of live cell imaging of the GFP-MG53 movement process can be found in Supplementary Movie 1 . ( b ) RLE cells were treated with external rhMG53 or boiled rhMG53 (denatured control protein) in the cell culture medium and then exposed to mechanical membrane damage by glass beads. Membrane damage is measured by LDH release from cells. rhMG53 reduced LDH release due to mechanical damage and this protective effect is dose dependent, n =9–12 for each data point (mean±s.e.m.). Full size image We previously showed that the rhMG53 protein can protect various cell types against cell membrane disruption when applied to the extracellular solution [19] . Here we examined whether rhMG53 was effective in protecting RLE cells from mechanical injuries. As shown in Fig. 3b , application of rhMG53 to the extracellular solution before RLE cells were injured with glass micro-beads [8] , [11] , [19] reduced the amount of intracellular enzyme, lactate dehydrogenase (LDH), released from the cells into the culture medium in a dose-dependent manner. Reduced LDH release from RLE cells indicates that there was decreased membrane disruption. As control, denatured rhMG53 protein proved to be ineffective at minimizing membrane damage in this assay. Our previous study demonstrated that the membrane repair function for rhMG53 was mediated by interaction with exposed phosphatidylserine at the injury sites [19] . To test whether this also occurs in the lung epithelial cells, we used the A549 human lung epithelial cells that were subjected to treatment with anoxia/reoxygenation (A/R). As shown in Fig. 4a , in A549 cells without treatment of A/R, the endogenous MG53 protein was mostly distributed in the cytosol (left panel); after A/R treatment, more MG53 was distributed at the cell surface membrane (right panel). The exogenously applied rhMG53 could concentrate at the cell surface membrane only in A/R-treated A549 cells but not in untreated cells ( Fig. 4b ). This membrane localization pattern appeared to be specific for rhMG53, as labelled BSA applied to the cells could not translocate to the injured membrane of A/R-treated A549 cells. Strong co-localization of labelled rhMG53 (Rhodamine red fluorescence) and Annexin V (fluorescein isithiocyanate (FITC) green fluorescence) at the surface membrane of A/R-treated A549 cells could be detected ( Fig. 4c ), indicating that the membrane repair effect of rhMG53 in lung epithelial cells is probabbly mediated through binding to phosphatidylserine at the injured surface membrane. 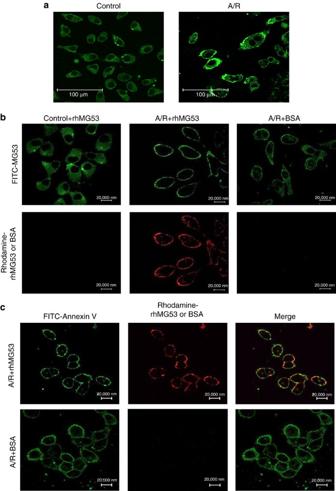Figure 4: Localization of MG53 to the surface membrane of A549 cells after treatment with anoxia and reoxygenation (A/R). (a) Immunofluorescence staining of endogenous MG53 in A549 cells. Control cells show cytosolic distribution of MG53- and A/R-treated cells display membrane localization of MG53. (b) Top panels show FITC staining of endogenous MG53 in control cells (left), A/R-treated cells (middle and right). Bottom panels show Rhodamine-labelled rhMG53 added to control cells (left) and A/R-treated cells (middle), or Rhodamine-labelled BSA added to A/R-treated A549 cells (right). (c) Left panels show FITC-labelling of Annexin V in A/R-treated A549 cells following incubation with rhMG53 (top) or BSA as control (bottom).Middle panels show Rhodamine-labelling of rhMG53 (top) or lack of Rhodamine-labelling of BSA (bottom) in A/R-treated A549 cells. Right panels show colocalization of Annexin V and rhMG53 (top) and lack of colocalization between Annexin V and BSA (bottom) in A/R-treated A549 cells. The images shown were representative of >104cells in at least four separate experiments. Figure 4: Localization of MG53 to the surface membrane of A549 cells after treatment with anoxia and reoxygenation (A/R). ( a ) Immunofluorescence staining of endogenous MG53 in A549 cells. Control cells show cytosolic distribution of MG53- and A/R-treated cells display membrane localization of MG53. ( b ) Top panels show FITC staining of endogenous MG53 in control cells (left), A/R-treated cells (middle and right). Bottom panels show Rhodamine-labelled rhMG53 added to control cells (left) and A/R-treated cells (middle), or Rhodamine-labelled BSA added to A/R-treated A549 cells (right). ( c ) Left panels show FITC-labelling of Annexin V in A/R-treated A549 cells following incubation with rhMG53 (top) or BSA as control ( bottom). Middle panels show Rhodamine-labelling of rhMG53 (top) or lack of Rhodamine-labelling of BSA (bottom) in A/R-treated A549 cells. Right panels show colocalization of Annexin V and rhMG53 (top) and lack of colocalization between Annexin V and BSA (bottom) in A/R-treated A549 cells. The images shown were representative of >10 4 cells in at least four separate experiments. Full size image Intravenous delivery of rhMG53 ameliorates I/R-induced lung injury Given the protective effects seen with rhMG53 in RLE and A549 cells, we tested whether systemic application of rhMG53 can protect against I/R-induced lung injury in vivo . Based on the in vitro assay using rhMG53 in RLE cells ( Fig. 3b ), we determined a dose of 6 mg rhMG53 protein per kg body weight for experiments with the rat model. This dose was applied by intravenous (IV) injection through the tail vein 30 min before the animals were subjected to I/R-induced lung injury. To quantify the effect of rhMG53 on I/R-induced lung oedema, the wet/dry ratio was measured ( Fig. 5a ). Clearly, rhMG53 application produced a significant reduction in oedema compared with the control group. Hypoxaemia is another pathologic change after lung I/R injury. Arterial blood gas analysis showed that PaO 2 was decreased in the I/R-treated group relative to the sham-operated group, and application of rhMG53 significantly improved PaO 2 function in rats subjected to I/R lung injury ( Fig. 5b ). Although the concentration of pro-inflammatory cytokines (interleukin (IL)-1β and IL-6) in the serum were elevated in rats subjected to I/R lung injury, the application of rhMG53 led to significant reduction in these pro-inflammatory factors ( Fig. 5c,d ). 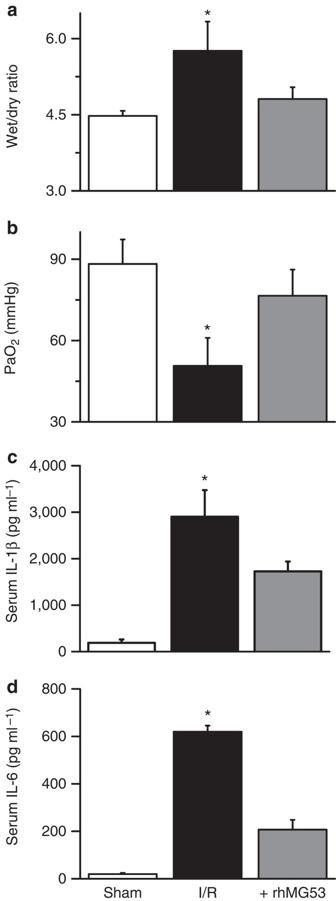Figure 5: Protective effect of rhMG53 against I/R-induced lung injury in rats. (a) Effect of rhMG53 precondition on oedema in lung from I/R rats. Lung oedema was measured as the wet/dry weight ratio of the excised lung tissue from rats (*P<0.05 versus others,n=5, analysis of variance (ANOVA), mean±s.e.m.). (b) Effect of rhMG53 precondition on gas exchange after I/R. Arterial blood samples were drawn from individual rats, the plasma PaO2concentrations were measured (*P<0.05 versus others,n=6 in each group, ANOVA, mean±s.e.m.). (c,d) Effect of rhMG53 precondition on serum IL-1β and IL-6 concentrations in I/R-injured Sprague–Dawley (SD) rats. Serum levels of IL-1β (c) and IL-6 (d) were measured by enzyme-linked immunosorbent assay (*P<0.05 versus others,n=5, ANOVA, mean±s.e.m.). Figure 5: Protective effect of rhMG53 against I/R-induced lung injury in rats. ( a ) Effect of rhMG53 precondition on oedema in lung from I/R rats. Lung oedema was measured as the wet/dry weight ratio of the excised lung tissue from rats (* P <0.05 versus others, n =5, analysis of variance (ANOVA), mean±s.e.m.). ( b ) Effect of rhMG53 precondition on gas exchange after I/R. Arterial blood samples were drawn from individual rats, the plasma PaO 2 concentrations were measured (* P <0.05 versus others, n =6 in each group, ANOVA, mean±s.e.m.). ( c , d ) Effect of rhMG53 precondition on serum IL-1β and IL-6 concentrations in I/R-injured Sprague–Dawley (SD) rats. Serum levels of IL-1β ( c ) and IL-6 ( d ) were measured by enzyme-linked immunosorbent assay (* P <0.05 versus others, n =5, ANOVA, mean±s.e.m.). Full size image In Supplementary Fig. 3 , we show that the IV-injected rhMG53 appeared in the bronchial alveolar lavage fluid (BALF) following lung injury, and rhMG53 protein could associate with both lung alveolar cells and endothelial cells to protect against stress-induced injury to the lung. It is known that oedema in ALI is a consequence of increased permeability of the alveolar–capillary barrier, the protective effect of rhMG53 against damage to both alveolar epithelial and endothelial cells could contribute to the improved pulmonary function in animals treated with rhMG53. To support this conclusion, we show in Supplementary Fig. 4 that the levels of IL-1β and IL-6 in the BALF were significantly reduced with rhMG53 administration, and I/R-induced elevation of HSP70 was also ameliorated by rhMG53 administration. The above studies show the prophylactic effect of rhMG53 in prevention of I/R-induced lung injury. To test whether rhMG53 has therapeutic value for treatment of ALI, we intravenously injected rhMG53 to rats either immediately before reperfusion or at 0.5 h after reperfusion. The data shown in Supplementary Fig. 5 showed that application of rhMG53 at either of these times could ameliorate I/R-induced injury to the lung tissue, as both wet/dry weight ratio and PaO 2 measurements were restored close to the sham-operated animal group. In addition, serum IL-1β and IL-6 concentrations were lower in rhMG53 treatment group. We performed histopathological analyses to evaluate the changes in lung structure following I/R injury with or without rhMG53 treatment. These analyses were quantified in a blinded manner using standard methods established by Takil et al. [25] , as outlined in Supplementary Table 2 . As shown in Supplementary Fig. 6a , lung sections in the sham group displayed normal alveolar architecture, whereas the lung sections in the I/R group showed obvious oedema, haemorrhage, extensive alveolar wall disruption and a great number of infiltrating inflammatory cells in the interstitium and alveoli. These symptoms were alleviated with rhMG53 administration. Data from multiple experiments are summarized in Supplementary Fig. 6b , which illustrates that pulmonary protective effects of rhMG53 were observed under all three paradigms of rhMG53 application, for example, precondition, treatment and 0.5-h treatment. The pulmonary protective effect of rhMG53 was further examined in the mg53−/− mice following I/R lung injury. These results are summarized in Supplementary Fig. 7 . Consistent with the data obtained with the rat model, we found that rhMG53 administration into the mg53−/− mice after I/R-induced lung injury could improve the survival rate, wet/dry ratio and blood gas exchange function. Intratracheal delivery of rhMG53 protects against PPE-induced lung injury We next used an enzyme-induced emphysema rat model to examine whether intratracheal (i.t.) delivery of rhMG53 can produce beneficial effects on the structure and function of the lung following acute injury. In this model, rats were treated with the porcine pancreas elastase (PPE, 500 U kg −1 ) by i.t. spray to produce damage to the airway epithelial lining [26] . As shown in Fig. 6a , 30 min after PPE application, LDH levels in BALF was significantly increased, indicating that the plasma membrane of the airway epithelium was damaged by PPE. Intratracheal application of rhMG53 at 5 min before PPE decreased this LDH release into BALF in a concentration-dependent manner. Denatured rhMG53 (boiled for 20 min) or BSA was ineffective at alleviating PPE-induced LDH release, suggesting rhMG53 can prevent PPE-induced acute cell damage to the airway epithelium. 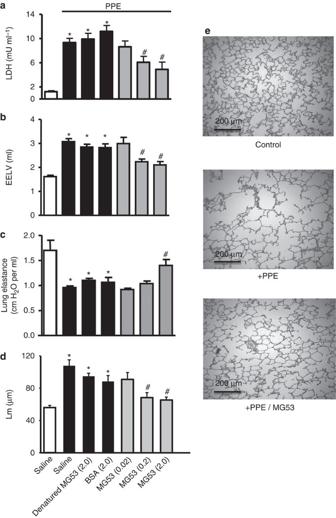Figure 6: Intratracheal (i.t.) instillation of rhMG53 protects PPE-induced injury to rat lung. (a) PPE was applied through i.t. spray. LDH in BALF was measured 30 min after PPE application to evaluate cell damage. Different concentrations of MBP-MG53 or control proteins (denatured MBP-MG53 or BSA) were applied through i.t. spray 5 min before PPE. 0.2 and 2 mg kg−1MBP-MG53 significantly reduced LDH in BALF. The measurements of chronic responses were conducted 4 weeks after PPE application with repetitive application of MBP-MG53 (i.t., 5 days per week for 4 weeks). EELV (b), lung elastance (c) and alveolar structure (quantified by Lm) of the lung (d) were compared with control treatment groups.n=7–10 per group. (e) Representative histology images of lung parenchyma in PPE-induced injury to rat lung with or without administration of MG53 (scale bars, 200 μm). *P<0.05 versus saline control group (open bar).#P<0.05 versus denatured MBP-MG53 group (Mann–WhitneyU-analysis). Figure 6: Intratracheal (i.t.) instillation of rhMG53 protects PPE-induced injury to rat lung. ( a ) PPE was applied through i.t. spray. LDH in BALF was measured 30 min after PPE application to evaluate cell damage. Different concentrations of MBP-MG53 or control proteins (denatured MBP-MG53 or BSA) were applied through i.t. spray 5 min before PPE. 0.2 and 2 mg kg −1 MBP-MG53 significantly reduced LDH in BALF. The measurements of chronic responses were conducted 4 weeks after PPE application with repetitive application of MBP-MG53 (i.t., 5 days per week for 4 weeks). EELV ( b ), lung elastance ( c ) and alveolar structure (quantified by Lm) of the lung ( d ) were compared with control treatment groups. n =7–10 per group. ( e ) Representative histology images of lung parenchyma in PPE-induced injury to rat lung with or without administration of MG53 (scale bars, 200 μm). * P <0.05 versus saline control group (open bar). # P <0.05 versus denatured MBP-MG53 group (Mann–Whitney U -analysis). Full size image The elastase-induced rat model of emphysema allowed us to further probe whether the protective effect of rhMG53 on the acute tissue injury can be translated into long-term improvement in the structure and function of the lung. Chronic treatment with rhMG53 in rats subjected to PPE-induced lung injury was conducted with daily application of rhMG53 for 4 weeks. By 4 weeks after PPE application, this model develops several emphysema-related changes [41] . Accordingly, end expiratory lung volume (EELV) increased from 1.62±0.06 to 3.07±0.13 ml and lung elastance decreased from 1.70±0.21 to 0.96±0.03 cm H 2 O per ml in PPE-treated rats. rhMG53 treatment significantly attenuated PPE-induced functional changes in a dose-dependent manner ( Fig 6b,c ). When animals were treated with 2 mg ml −1 rhMG53, EELV was attenuated to 2.10±0.14 ml and the lung elastance was maintained at 1.40±0.12 cm H 2 O per ml ( Fig 6b,c ). These rats displayed significant enlargement of the alveolar space, which was partially attenuated by application of rhMG53 ( Fig. 6e ). The linear mean (Lm) intercept distance in the control group was 56.0±2.7 μm, which increased to 107.8±7.3 μm in the PPE group ( P <0.05 compared with the control group, Mann–Whitney U -analysis). Mean Lm in the PPE plus MG53 group (65.3±3.6 μm) was significantly smaller than in the PPE group ( P <0.05, Mann–Whitney U -analysis) ( Fig. 6d ). These data suggest that i.t. delivery of rhMG53 could have beneficial effect on structure and functional changes in the lung associated with emphysema. Intratracheal delivery of rhMG53 protects LPS-induced injury to the lung The effect of rhMG53 in prevention of chronic injury to the lung was further evaluated using a model of emphysema involving i.t. application of lipopolysaccharide (LPS; 0.2 mg ml −1 ) in C57BL/6J mice [27] . Mice were treated with LPS three times a week for 4 weeks. All animals were housed for another week before the measurements of emphysema-related changes. As shown in Fig. 7a , the whole mount specimen of lungs from mice treated with LPS demonstrated bullae on the lung surface, a typical pathological change in emphysema. Remarkably, injecting mice with rhMG53 prevented the appearance of LPS-induced bullae on the lung surface. Histological examination showed expected levels of airspace enlargement and disrupted alveolar septa in LPS-treated mice. These changes were greatly reduced by rhMG53 treatment ( Fig. 7b ). 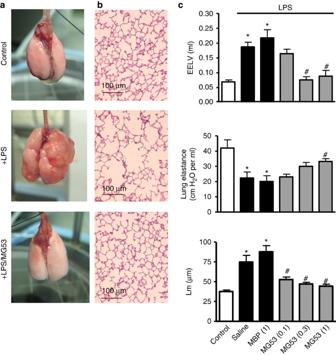Figure 7: Intratracheal application of rhMG53 protects LPS-induced lung remodelling in mice. Animals were first treated with LPS (i.t., 3 times per week, for 5 weeks) followed by MBP-MG53 or MBP–MBP in control group (i.t., 5 days/week for 5 weeks). Lungs were collected 5 weeks after initial LPS application for evaluation. (a) MBP-MG53 prevents emphysema in LPS-induced chronic lung remodeling. (b) Histology haematoxylin and eosin staining of parenchyma in LPS-induced emphysematous lung (scale bars, 100 μm). (c) Statistical results for EELV, lung elastance and Lm in LPS-induced emphysematous lung treated with different doses of rMG53 (mg kg−1, 0.1, 0.3, 1.0) and 1 mg per kg control protein,n=7–10, *P<0.05 compared with no LPS control group (open bar) and#P<0.05 compared with saline-treated, LPS-challenged group.n=7–10 (Mann–WhitneyU-analysis). Figure 7: Intratracheal application of rhMG53 protects LPS-induced lung remodelling in mice. Animals were first treated with LPS (i.t., 3 times per week, for 5 weeks) followed by MBP-MG53 or MBP–MBP in control group (i.t., 5 days/week for 5 weeks). Lungs were collected 5 weeks after initial LPS application for evaluation. ( a ) MBP-MG53 prevents emphysema in LPS-induced chronic lung remodeling. ( b ) Histology haematoxylin and eosin staining of parenchyma in LPS-induced emphysematous lung (scale bars, 100 μm). ( c ) Statistical results for EELV, lung elastance and Lm in LPS-induced emphysematous lung treated with different doses of rMG53 (mg kg −1 , 0.1, 0.3, 1.0) and 1 mg per kg control protein, n =7–10, * P <0.05 compared with no LPS control group (open bar) and # P <0.05 compared with saline-treated, LPS-challenged group. n =7–10 (Mann–Whitney U -analysis). Full size image LPS treatment increased the mean linear intercept (Lm) and EELV from 37.5±2.0 μm and 69±6 μl to 74.7±8.5 μm and 187±16 μl, respectively ( Fig. 7c ). LPS also decreased lung elastance from 42.0±5.4 cm H 2 O per ml to 22.4±3.9 cm H 2 O per ml. Treating these animals with rhMG53 (0.1–1.0 mg ml −1 , i.t. 5 weeks) significantly improved the pathological changes. In the MG53 treatment group (1.0 mg ml −1 ), the value of Lm, EELV and lung elastance are 44.4±2.5 μm, 88±19 μl and 33.2±1.8 cm H 2 O per ml, respectively. These results provide direct evidence that rhMG53 restored emphysema-related morphological and functional changes in the LPS-induced emphysema model in mice. The data presented in this study are consistent with the hypothesis that MG53-mediated cell membrane repair contributes to the normal physiology function of the lung, and that defects in membrane repair due to the absence of MG53 can lead to increased susceptibility of the lung to stress-induced injury. We also present evidence that application of the exogenous rhMG53 protein have beneficial effects in treatment or prevention of lung injury in various animal model systems. As our previously published studies with MG53 function in cell membrane repair were mostly conducted in skeletal and cardiac muscles [5] , [6] , [7] , [9] , [10] , [28] , the observation of MG53 expression in the lung tissue is novel. Using RACE analysis, we found that the mRNA coding sequence for mg53 in the lung is identical to that in muscle cells, suggesting that the mg53 gene expresses one product in both tissues without alternative splicing. Interestingly, there is a slight mobility change of MG53 in the lung tissue compared with that in the muscle tissue. Further efforts will be required to test whether this apparent shift in mobility was related to the differential post-translational mechanisms that may exist in these two tissues. The cell membrane in lung epithelial cells and striated muscle cells are both exposed to mechanical stresses during the course of normal physiology. These cell types constantly undergo stretch or deformation-induced injury in the course of their function in their resident tissue. Even though the level of MG53 protein in the lung tissue is substantially less than that in the muscle cells, a clear lung phenotype was observed with the mg53−/− mice under stress conditions, as these animals are vulnerable to I/R- and overventilation-induced injury to the lung. Based on immunoblotting and histological studies, we show that MG53 is present in both type I and type II alveolar cells, but absent from endothelial cells. The lung epithelium represents an important barrier that protects the internal organs from exposure to external environment. Although normal tidal breathing produces little mechanical strain across alveolar cells, overventilation may cause stress to the lung and lead to injury to alveolar cells [29] . In pathophysiological settings such as mechanical ventilation, I/R injury, sepsis, trauma and shock, these insults can lead to damage to the organ. If the injured lung epithelial cells cannot repair, an excessive pro-inflammatory response may occur in the lung and trigger a cascade of detrimental events leading to extensive damage of the lung and eventual failure of pulmonary function. Targeting repair of cell membrane injury has recently emerged as an attractive avenue for prevention and/or treatment of ALI. Several studies have demonstrated protective effect for P188, a polymer with membrane sealing capacity, against injury to spinal cord [30] , [31] and heart [32] , [33] . A previous study by Plataki et al. [24] showed that P188 has protective effect in cultured lung epithelial cells from stretch-induced injury. However, this protective effect of P188 can only be seen in isolated perfused lungs but not in living rats subjected to overventilation for reasons that are currently unknown [24] . Compared with P188, rhMG53 has several advantages for treatment of cell membrane injuries. MG53 is an intrinsic tissue-repair gene present in the human body, and the primary amino acid sequence of MG53 is highly conserved among various animal species. Native MG53 protein is constantly present in blood circulation due to tissue injury, thus reducing the potential immunogenic responses associated with systemic delivery [19] . Our published data showed that rhMG53 is effective at facilitating cell membrane repair at lower concentrations than P188. Thus, targeting MG53-mediated membrane repair in lung epithelial cells could potentially be an effective and integrative component of ALI therapies. The therapeutic effect of rhMG53 on ALI was assessed in two different rodent models of emphysema involving tracheal application of LPS or elastase. Chronic administration of LPS in the airway probably induces airway inflammation and emphysematous-related changes through endogenous inflammatory mediators, which induce oxidant stress, protease/antiprotease imbalance and apoptosis [27] , [34] . This model resembles some of the changes seen in human emphysema [35] , although the mechanisms at work in the model are not clearly defined. The elastase-induced emphysema results from destruction of lung parenchyma tissues. Such models have been widely used to evaluate pharmacological effect on emphysema targeting lung regeneration [36] , [37] . In both experimental models of emphysema, we showed that rhMG53 could significantly attenuate the emphysema-related changes including air space enlargement, loss of lung elastance and elevation of EELV when compared with that in vehicle control-treated animals. As lung elastic recoil property is the driving force for expiration, loss of lung elastic recoil function in the emphysematous lungs leads to expiratory air flow limitation and chronic lung hyperinflation, that is known to play a significant role in the development of dyspnoea and exercise limitation that are major clinical manifestations of chronic obstructive pulmonary disease [38] . Our studies with the rodent animal models show that IV as well as i.t. delivery of rhMG53 are both effective in protecting injury to the lung epithelial cells and restoring the pulmonary function following ALI. Although i.t. delivery of rhMG53 can be conveniently achieved through nebulization, further formulation efforts will be needed to efficiently target the lower airway epithelial cells to increase the potential efficacy for rhMG53 in treatment or prevention of ALI. The systemic delivery of rhMG53 via IV route is potentially an attractive avenue for treatment of ALI, especially for patients with more severe pulmonary dysfunction. We have previously shown that IV delivery of rhMG53 does not produce overt toxicity in rodent models [19] . Here we find that IV application of rhMG53 can have protective effects against I/R-mediated acute injury to the lungs. Overall, we provide evidence that injury to lung resident cells is involved in the pathogenesis of acute and chronic lung diseases, and targeting lung cell repair represents a novel disease-modifying treatment for ALI. Future studies should focus on understanding the mechanism for MG53-mediated repair, for example, identification of co-factors that participate in the nucleation process of membrane repair in pulmonary cells. Moreover, elucidating the mechanism of action for the exogenous rhMG53 protein in protection of ALI should improve the potential of rhMG53 as a therapeutic agent for treatment of ALI. Immunoblotting and RACE analysis Isolated lung tissues were washed twice with ice-cold PBS and lysed in lysis buffer (10 mM Tris-HCl, pH 8.0, 150 mM NaCl, 1% NP-40, 1 mM phenylmethylsulphonyl fluoride and 10 mg ml −1 each leupeptin and aprotinin). After centrifugation at 12,000 g for 15 min, the supernatants were collected and their protein concentrations measured. The lung tissue homogenates (50 μg of protein) were separated by 10% SDS–PAGE and transferred onto polyvinylidene fluoride membranes (Bio-Rad). For quantification purpose, different amounts of skeletal muscle tissue lysates were loaded into the same gel. The blots were washed with Tris-buffered saline Tween-20, blocked with 5% milk in Tris-buffered saline Tween-20 buffer for 1 h and incubated with custom-made rabbit monoclonal anti-MG53 and the appropriate secondary antibody coupled to horseradish peroxidase (Sigma, 1:5,000 dilution). Bands were visualized with an ECL+ kit (Pierce). The amount of protein transferred onto the polyvinylidene fluoride membranes was verified by Ponceau S staining. RACE was conducted using a mouse lung Marathon-Ready cDNA library purchased from Clontech (catalogue number 639411). The primer sequences used for 5′-RACE and 3′-RACE were listed in Supplementary Table 1 . RACE amplifications were performed in 20 μl reaction volume using 2 μl mouse lung cDNA, 0.3 μM primers, 0.4 mM dNTPs and 0.4 unit of KOD Fx (TOYOBO, Japan). Conditions were as follows: 94 °C for 2 min; 5 cycles of 98 °C for 10 s and 74 °C for 2 min; 5 cycles of 98 °C for 10 s and 72 °C for 2 min; and 30 cycles of 98 °C for 10 s and 70 °C for 2 min, and 72 °C for 5 min. PCR products were subcloned into pBS-SK vector (Stratagene) and sequenced. Isolation and administration of recombinant human MG53 protein Purification of the rhMG53 protein has been described previously [19] . The present study employed two different forms of MG53 protein, MBP-MG53 and untagged rhMG53. MBP-MBP control proteins contained two copies of the MBP (maltose-binding protein) tag attached in tandem and were isolated by identical purification methods. Untagged rhMG53 was produced by cleavage of MBP from MBP-MG53 using thrombin and separation of these two using gel filtration high-pressure liquid chromatography. Untagged rhMG53 was lyophilized and stored at 4 °C as dry powder in a desiccator. For IV injection of rhMG53, the protein was diluted in 0.9% sterile saline, filtered through a 0.2-μm filter and injected via the tail vein. For i.t. application of rhMG53, animals were placed under anaesthesia (2–5% isoflurane, inhaled in a chamber) and the protein was applied into the trachea, using a laryngoscope and a micro sprayer (Penn-Century Inc., Philadelphia, PA). Cell culture and in vitro membrane injury assays The RLE cells, human primary pulmonary artery endothelial cells and umbilical vein endothelial cells were all obtained from American Type Culture Collection (Manassas, VA) and the standard culture conditions were followed accordingly. Human lung microvascular endothelial cells were purchased from Lonza (Alpharetta, GA). For in vitro membrane injury assays, RLE cells were cultured in F-12 culture medium supplemented with 10% fetal bovine serum and 1% penicillin/streptomycin. Transfection of GFP-MG53 into RLE cells was performed using the Lipofectamine LTX reagent (Life Technologies) as per the manufacturer’s instructions. RLE cells expressing GFP-MG53 was subjected to microelectrode penetration-induced acute injury to the plasma membrane as previously described [5] . Micro-glass beads-induced injury to RLE cells in suspension was conducted according to our published protocol [8] , [11] , [19] . Cells (9 × 10 4 ) were suspended in 150 μl of PBS in the presence or absence of acid washed beads, and/or different concentrations of rhMG53 in a 96-well plate. The plate was shaken on a rotary orbital shaker (Belloco Biotechnology) at 180 r.p.m. for 6 min at room temperature. After shaking, the cells were immediately centrifuged at 1,000 g for 5 min and 50 μl of supernatant was transferred into a new 96-well plate. LDH activity in this supernatant was determined using a LDH Cytotoxicity Detection kit (Takara Bio Inc.). Animal care Animal handling and surgical procedure was performed in accordance with local regulations and all protocols were approved by all participating Institutional Animal Care and Use Committee, including The Ohio State University, Daping Hospital-The Third Military Medical University and Schering-Plough Research Institute-Merck Research Labs, and were compliant with the guidelines of the American Association for the Accreditation of Laboratory Animal Care. MG53 knockout mice ( mg53−/− ) and their wild-type control mice were breed and maintained as previously described [5] . All other animals were obtained from commercial sources indicated for each procedure. Overventilation-induced lung injury and BALF collection The study protocol was approved by the Institutional Animal Care and Use Committee of the Ohio State University. Wild-type and mg53−/− mice [5] were anaesthetized with isoflurane and then overventilated at 30 ml kg −1 (Harvard Apparatus) for 30 min. For animals in the imaging study group, PI (1 μg ml −1 ) (Invitrogen, Eugene, OR) was administered into the right ventricle immediately after cessation of the mechanical ventilation, and ex bloc lung was occluded at peak inspiration for confocal imaging of the subpleural lung area. Positive end-expiratory pressure was not used for these studies. Cell membrane injury was expressed as a ratio of the number of PI-positive cells per total number of alveoli in the field from eight random subpleural images. In separate experiments, rhMG53 (2 mg kg −1 ) were administered via IV injection into mg53−/− mice immediately before overventilation-induced ALI described above. The BALF was collected and immunoblotting used for detection of rhMG53 in the BALF. Assessment of rhMG53 effects on I/R-induced lung injury in rats Sprague–Dawley rats of both sexes, weighing 210–250 g, were obtained from the Experimental Animals Centre of Daping Hospital at Chongqing, China. The experimental procedure for I/R-induced ALI was conducted according to published protocols with minor modifications [39] , [40] , [41] . Rats were randomized into sham-operated, and lung I/R groups with or without rhMG53 treatment. Rats were anaesthetized with an intraperitoneal injection of sodium pentobarbital (50 mg kg −1 ) and placed on a heating pad to maintain their body temperature. The right femoral arteries and vein of rats were then catheterized with polyethylene tubing (outer diameter=0.965 mm; inner diameter=0.58 mm) for arterial blood sampling and rhMG53 (or saline as control) injection. After intubation via tracheotomy, rats were placed on a volume ventilator (tidal volume=6 ml kg −1 , respiratory rate=60 breaths per minute, inspiratory/expiratory ratio=1: 2) with room air. After thoracotomy, the left hilum of I/R group was clamped for 1 h and released for reperfusion for 1 h. The left lungs were observed for atelectasis and inflation to make sure of adequate hilum clamping and reperfusion. The sham group underwent thoracotomy and was placed on ventilator without left hilum clamp. Rats that underwent I/R procedures were further divided into the following subgroups: untreated ‘I/R’ group; rhMG53 ‘precondition’ group—rhMG53 was administered in between thoracotomy and ischaemia; rhMG53 ‘treatment’ group—rhMG53 was administered immediately after 1 h ischaemia but before reperfusion; and rhMG53 ‘0.5 h treatment’ group—rhMG53 was administered 0.5 h after reperfusion. After reperfusion, blood samples were obtained immediately for arterial blood gas analysis (Gem primer 3000, Instrumentation Laboratory, US) and serum collection for enzyme-linked immunosorbent assay measurement of IL1β and IL6 (Boster, Wu Han, China). I/R-induced lung injury in mice followed the same protocol as that used for rats, with the following modifications. mg53−/− and wild-type mice (3–4 months) were connected to a Harvard ventilator (Hugo Sachs Elektronik, German) with an inspiratory pressure of 7 ml kg −1 after anaesthetization with sodium pentobarbital and intubation via tracheotomy (normal low-tidal ventilation). The respiratory rate was set at 100 breaths per minute. After thoracotomy, the left hilum of the I/R group was clamped for 1 h, and released, reperfusion proceeded for 1 h. Histological analysis and wet/dry ratio determination The left lung from Sprague–Dawley rats and mice were washed with ice-cold oxygenated saline to remove blood and then fixed in 4% neutral-buffered paraformaldehyde for 1–2 days at 4 °C before processing for paraffin embedding. Blocks were sectioned (4 μm), mounted on slides, then deparaffinized and rehydrated by successive incubations in xylene, 100% ethanol, 95% ethanol, 75% ethanol and PBS. Sections were stained with haematoxylin and eosin using standard procedures and scored according to a four-point scale [25] by an experienced histologist from the Department of Pathology at Daping Hospital under blinded conditions. The histological analyses were performed in ten randomly selected microscope fields ( × 200) from each section. Fresh lungs from separate groups of mice or rats were weighed and then desiccated until a stable dry weight was achieved. To measure the wet lung, the left lungs of rats and mice were weighted immediately after dissection. To measure dry weight, the tissues were desiccated then placed in an oven at 80 °C for 24 h and re-weighted as a dry weight for calculation of the wet/dry weight ratio. Anoxia and reoxygenation induced injury in A549 cells A549 cells were obtained from the American Type Culture Collection. To induce anoxia, cells were placed in an anoxic chamber with 5% CO 2 and 95% N 2 at 37 °C for 2 h followed by reoxygenation for 2 h. Exogenous rhMG53 was conjugated with Rhodamine by a dye labelling kit (G-Biosciences, St Louis, USA) and applied to cells immediately after anoxia. After the reoxygenation period, the cells were used for Annexin V staining or immunofluorescence staining. Cells were fixed with 4% paraformaldehyde (30 min) and custom rabbit anti-MG53 antibody was applied (1:200 dilution) overnight at 4 °C, which was followed by FITC-conjugated goat anti-rabbit IgG antibody (Jackson ImmunoResearch Laboratory, West Grove, PA). Immunofluorescence confocal images were acquired (Olympus AX70 laser confocal microscopy) at excitation wavelengths of 350 and 507 nm; emission was detected at 450 and 529 nm. Cells that were treated with only FITC-conjugated goat anti-rabbit IgG antibody revealed no immunofluorescence and omission of the anti-MG53 antibody showed no green fluorescence after merging the images. Intratracheal PPE- or LPS-induced emphysema models in rodent Emphysema animal models were induced as described previously [27] , [36] . Emphysema was induced in Wistar rats by one time i.t. application of PPE (500 U kg −1 , Elastin Products Co., Owensville, MO), using a laryngoscope and a micro sprayer (Penn-Century Inc., Philadelphia, PA), under anaesthesia by 2–5% isoflurane (inhaled in a chamber). MG53 or control proteins were applied intratracheally using the same method, 5 days per week for 4 weeks, starting on the day of PPE application. The emphysema-related changes were evaluated 4 weeks after the PPE application [36] . Emphysema was also induced in mice by LPS (Sigma-Aldrich, Saint Louis, Missouri) as described [27] . Briefly, animals under anaesthesia (2–5% isoflurane, inhaled in a chamber) was applied with LPS (i.t. application in mice: 0.2 mg ml −1 , 50 μl per animal) into the trachea, using a laryngoscope and a micro sprayer (Penn-Century Inc.), 3 times a week for 5 weeks. MBP-MG53, or MBP–MBP in the control group, was applied into the trachea once daily, 5 days a week for 5 weeks, starting on the first day of the LPS application. All the measurements were conducted 5 weeks after initial LPS application. EELV was measured ex vivo according to Borzone et al. [42] Briefly, rats or mice were killed and trachea was occluded at the end of expiration with the chest wall intact. The lungs with the occluded trachea were then removed and the whole lung volume was estimated by saline solution volume displaced by the isolated lungs. The lung tissue volume was estimated by lung tissue weight divided by tissue density. EELV was calculated as the difference between the whole lung volume and the lung tissue volume. Here we used the water density (1 g ml −1 ) to estimate lung tissue density as described previously [38] , [39] , [40] . The true tissue density may be greater than water density (for example, fat/water free liver density is 1.4 g ml −1 (refs 39 , 40 )). In addition, the saline on the surface of lung tissues cannot be completely excluded from the lung weight measurements. These factors may overestimate lung tissue volume and thus underestimate EELV. However, these systemic error applies to all the groups equally and do not affect the comparisons among groups. Static deflationary volume–pressure relationship was determined in isolated lungs to assess the lung elastic properties according to Borzone et al. [42] Briefly, immediately after isolation, the lungs were connected to a syringe filled with air and a differential pressure transducer through trachea. Transpulmonary pressure was measured as the i.t. pressure. The lungs were slowly inflated with air to 20 cm H 2 O twice. Step lung deflation maneuvres were performed. The i.t. pressure and the lung volume at each step were recorded after waiting for at least 10 s. The deflationary static volume–pressure curve of the lung was established, and the lung elastance at low lung volumes (transpulmonary pressure of 0–5 cm H 2 O) was calculated as ( P 5 cmH 2 O − P 0cmH 2 O ) / ( V 5 cmH 2 O − V 0cmH 2 O ) , where P is the transpulmonary pressure and V is the lung volume. The isolated lungs were fixed with 10% formalin through trachea at a constant pressure of 20 cm H 2 O. The lung tissue was processed, sliced and stained with haematoxylin and eosin. An image from the same area in the right middle lobe of the lung was chosen for measurements of mean linear intercept (Lm). Three lines of equal distance on each image were analysed and Lm was calculated as the length of each line divided by the number of alveolar septum on the line. Lm was expressed as mean value analysed from the three lines. Statistical analysis The data are expressed as mean±s.e.m. Comparison within groups was made by Student’s t -test when comparing two experimental groups and by analysis of variance for repeated measures. Comparison among groups was made by analysis of variance with Holm–Sidak test. The product limit (Kaplan–Meier) estimate of the cumulative survival was assessed with the log-rank test to evaluate significance differences. A value of P <0.05 was considered significant. A subset between group comparisons employed a Mann–Whitney U -statistical analysis. The statistical significance level was set at P <0.05 or P <0.01 as specified in figure legends. How to cite this article: Jia, Y. et al. Treatment of acute lung injury by targeting MG53-mediated cell membrane repair. Nat. Commun. 5:4387 doi: 10.1038/ncomms5387 (2014).